Extreme surface propensity of halide ions in water Water possesses an extremely high polarity, making it a unique solvent for salts. Indeed, aqueous electrolyte solutions are ubiquitous in the atmosphere, biology, energy applications and industrial processes. For many processes, chemical reactions at the water surface are rate determining, and the nature and concentration of the surface-bound electrolytes are of paramount importance, as they determine the water structure and thereby surface reactivity. Here we investigate the dynamics of water molecules at the surface of sodium chloride and sodium iodide solutions, using surface-specific femtosecond vibrational spectroscopy. We quantify the interfacial ion density through the reduced energy transfer rates between water molecules resulting from the lowered effective interfacial density of water molecules, as water is displaced by surface active ions. Our results reveal remarkably high surface propensities for halogenic anions, higher for iodide than for chloride ions, corresponding to surface ion concentrations several times that of the bulk. In the past years, much progress has been made in the elucidation of the structure and dynamics of water molecules at the pure water–air interface [1] , [2] , [3] . However, the vast majority of water on earth is not pure water, but rather contains salts. Ions at the water–air interface are known to be particularly important for atmospheric chemistry [4] , [5] , [6] . At the surface of ion-containing aerosols, chemical reactions take place; if a surface propensity exists for dissolved ions, these will strongly affect the interfacial structure, dynamics and reactivity. This is especially true for seawater, which constitutes the bulk of the water reservoir present on earth, and from which salty aerosols are formed. Accordingly, many experimental and theoretical efforts have been aimed at elucidating the ion distribution at the interface of water. For the ubiquitous sodium halide salts, it has been established both through experiments [4] , [6] , [7] , [8] , [9] , [10] and molecular dynamics simulations [4] , [5] , [6] , [7] , [9] , [10] , [11] , [12] that, for example the Cl − ion has a weak, whereas the I − ion has a strong surface propensity. Moreover, a distinct spatial separation has been observed for ions at the water interface, with anions residing in the outmost surface layer, while cations occupying the subsurface region [4] , [13] , [14] , [15] , [16] , [17] . While the enhanced surface propensity of anions has been established qualitatively, it has been challenging to experimentally quantify the effective concentration of ions at the surface. Experimentally, synchrotron-based photoelectron spectroscopy (PES) experiments allow near-surface profiling of ions [13] , [14] , [18] , [19] . However, in one PES experiment, the surface concentration of iodide was observed to be ~2.5 times higher than the bulk concentration [14] , while in another, more recent PES experiment the surface iodide concentration was observed to be lower than the bulk concentration [13] . In both PES experiments, the electron energies were tuned such, that primarily the near-surface region was probed, but PES is not a purely surface-specific technique. Intrinsic surface specificity can be achieved using second-order non-linear optical probes of second harmonic generation (SHG) and sum frequency generation (SFG). The SHG and SFG intensities originate from the region of the solution where the centrosymmetric nature of the bulk solution is broken by the interface [20] . The precise SFG probing depth for surfaces of sodium chloride (NaCl) and sodium iodide (NaI) solutions has been determined by Ishiyama and Morita, by calculating the SFG spectrum as a function of the thickness of the surface layer considered in the calculation [15] . They found that the SFG spectrum no longer changes for thicknesses exceeding 6 Å, meaning that this value represents the maximum probing depth of the SFG experiment. A similar probing depth of ~5 Å has been found by Archontis et al . [16] The SFG probing depth (~6 Å) is smaller than the depth over which the ion concentrations vary (~12 Å) (refs 15 , 16 , 17 ), which can be understood by noting that the noncentrosymmetric region is not only determined by the depth at which the ion distribution equilibrates, but rather the depth at which a net water orientation vanishes. Water molecules that fully hydrate the subsurface ions possess a largely centrosymmetric solvation shell, and will thus not contribute to the SFG signal. It is thus safe to claim that mostly the outmost few (2–3) water layers will contribute to the SHG/SFG signal. SHG has been used to probe interfacial anions through their charge-transfer-to-solvent transitions in the UV [6] , but it has been intricate to separate the anion signal from the water signal, especially for halide anions, thus making it difficult to obtain quantitative information on the surface ion concentration. Static [8] and phase-resolved [9] SFG spectra clearly show that halide ions are present at the interface as spectral changes are observed on adding salts to water. However, these static SFG spectroscopies also do not allow for a direct quantification of the surface concentrations of these ions. Here, we use ultrafast, surface-specific SFG vibrational spectroscopy to determine the surface concentration of chloride and iodide ions. For experimental reasons, we study heavy water (D 2 O), rather than H 2 O (see Methods). We probe interfacial water molecules at the NaCl and NaI solutions-air interfaces. Through their presence at the interface, Cl − and I − displace water molecules and thereby alter the rate of resonant (Förster) vibrational energy transfer between water molecules at the interface, revealing anion surface concentrations approximately 1.8 and 3.5 times higher, respectively, than the bulk solution concentration. Static SFG spectroscopy In static SFG experiments, an infrared (IR) pulse is overlapped at the surface in both time and space with a visible (VIS) pulse. When the IR frequency is resonant with the OD stretch vibration of interfacial water, the sum frequency field generated by the interaction of the two pulses is strongly enhanced, with the SFG signal originating from the topmost few layers of water molecules at the air-water interface [20] . Exemplary SFG spectra (see Fig. 1 ) obtained from 3 M NaI/D 2 O (red), 3 M NaCl/D 2 O (green) and pure D 2 O (blue) interfaces show a broadband response at frequencies between 2350 and 2600 cm −1 , attributed to hydrogen-bonded OD groups, and a narrow peak at ~2750, cm −1 , attributed to free OD groups, sticking out of the liquid phase into the air. The SFG spectra shown in Fig. 1 are in agreement with previously reported static SFG spectra [8] , [9] , and show that the addition of ions affects the surface structure of water, which points to a surface propensity of the ions. With the addition of ions, the intensity of the free OD band decreases relative to that in the hydrogen-bonded region. Moreover, the hydrogen-bonded response shifts to the blue. This blueshift indicates a weakening of the hydrogen bonds at the surface, which agrees with the notion that hydrogen bonds between water molecules and anions are weaker than hydrogen bonds between water molecules. The blueshift is larger for NaI than for NaCl, which agrees with the fact that the strength of hydrogen bonds decreases within the halide ion series (F − >Cl − >Br − >I − ). 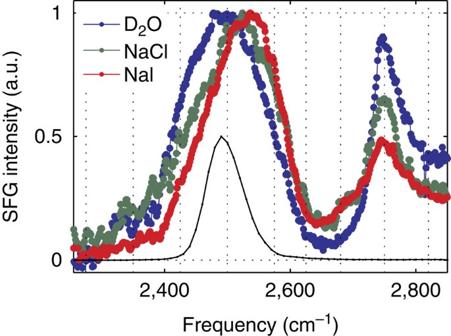Figure 1: Static SFG spectra of water and different salt solutions. SFG spectra recorded from the surfaces of 3 M solutions of NaI (red) and NaCl (green) and pure water D2O solutions (blue), normalized to the peak SFG intensity. An exemplary spectrum of the excitation pulse around 2500, cm−1is shown with a thin black line. Dashed lines indicate all the excitation frequencies used in the experiment. Figure 1: Static SFG spectra of water and different salt solutions. SFG spectra recorded from the surfaces of 3 M solutions of NaI (red) and NaCl (green) and pure water D 2 O solutions (blue), normalized to the peak SFG intensity. An exemplary spectrum of the excitation pulse around 2500, cm −1 is shown with a thin black line. Dashed lines indicate all the excitation frequencies used in the experiment. Full size image Time-resolved SFG spectroscopy We measure the vibrational energy relaxation dynamics of the OD groups at the surface of salt solutions using time-resolved IR-pump/SFG-probe spectroscopy [3] , [21] , [22] , [23] . In this technique, an IR excitation (pump) pulse excites OD groups at a specific vibrational frequency, and the effect of that excitation is followed in time with the SFG probe pair (for details see Methods). For the excited OD groups, the SFG intensity will temporarily be decreased (‘bleach’), and the recovery of the signal reflects vibrational relaxation. In Fig. 2a , we show the differential (SFG pump —SFG no_pump ) transient SFG spectra for a NaI solution excited at ~2500, cm −1 (excitation spectrum shown with the black line in Fig. 1 ). The SFG signal evolves in time and its maximum shifts towards lower frequency. After about 2.5 ps, the system reaches thermal equilibrium, which is reflected in the dispersive shape of the differential SFG signal that follows from the blueshift of the SFG response due to the heat released after vibrational relaxation. Inspecting the SFG signal after 5 ps we find that, subsequent to the fast vibrational relaxation dynamics, the SFG intensity undergoes slow, oscillatory changes on a timescale of hundreds of picoseconds. This oscillatory signal is the result of interference between the SFG signal reflected from the outer surface and that transmitted into the bulk, which is subsequently reflected from the wavefront of a pump-induced density wave propagating away from the interface. This additional signal has little effect on the short-time dynamics, and is readily corrected for. 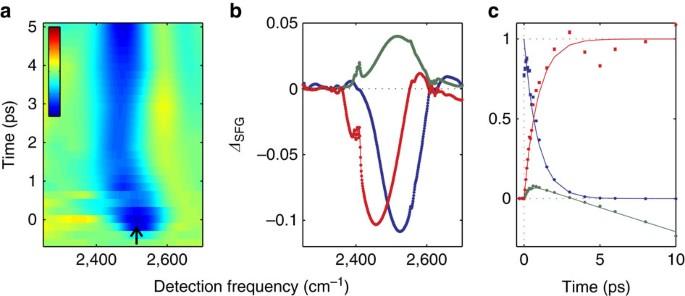Figure 2: Time-resolved SFG spectroscopy of the NaI solution surface. (a) Transient SFG spectra for a 3 M NaI solution (following excitation at 2500, cm−1, marked with an arrow) as a function of delay time between the excitation and detection pulses. Colourbar scale ranges from −0.2 to 0.2. (b) SFG spectra corresponding to a delay time of 1 ps, extracted from the global fit to the kinetic model described in the main text. The three spectra correspond to: excited vibrational state (blue), thermally equilibrated state (red) and spectral signature of the oscillatory signal (green). (c) Population dynamics associated with the states included in the model. Solid lines indicate dynamics of the kinetic model. Dots indicate time dynamics of the data reconstructed with the extracted spectra. Figure 2: Time-resolved SFG spectroscopy of the NaI solution surface. ( a ) Transient SFG spectra for a 3 M NaI solution (following excitation at 2500, cm −1 , marked with an arrow) as a function of delay time between the excitation and detection pulses. Colourbar scale ranges from −0.2 to 0.2. ( b ) SFG spectra corresponding to a delay time of 1 ps, extracted from the global fit to the kinetic model described in the main text. The three spectra correspond to: excited vibrational state (blue), thermally equilibrated state (red) and spectral signature of the oscillatory signal (green). ( c ) Population dynamics associated with the states included in the model. Solid lines indicate dynamics of the kinetic model. Dots indicate time dynamics of the data reconstructed with the extracted spectra. Full size image In order to extract the vibrational relaxation rate, we correct the data for the thermal and oscillatory signals (see Methods). In brief, we describe the data as a sum of three transient spectral components. Each of the spectral components is described as a product of its population dynamics and associated spectral signature. The three components represent: (1) the vibrational excited state, (2) the thermal state and (3) the oscillatory signal. From a global fit, we extract the spectra associated with each component. The spectra obtained at an excitation frequency of 2500, cm −1 are shown in Fig. 2b . The shape of the excited state spectrum (blue) follows closely the spectral shape of the excitation pulse. In Fig. 2c , we show the time-dependent populations of the three components. The model provides a very good description of all datasets, at all excitation and detection frequencies. Within the experimental resolution, the extracted vibrational lifetimes are independent of the excitation frequency, amounting to 1.35±0.2 ps and 1.4±0.2 ps for NaI and NaCl solutions, respectively. The extracted lifetimes are significantly longer than the vibrational lifetime of ~1 ps previously observed for interfacial D 2 O molecules at the water–air interface [2] . Given that sodium ions are not located at the interface, but rather in the subsurface layer [11] , [15] , [16] , [24] , we attribute this increase of the vibrational lifetime to interactions with anions, in analogy to the lifetime increase observed for water around negative ions in bulk salt solutions [25] , [26] , [27] , [28] . The slowdown of the vibrational relaxation can be understood from the weaker hydrogen bonds to the anion compared with water [25] , [26] , [27] , [28] . Rapid resonant (Förster) energy transfer between OD groups (see below) makes the measured lifetime frequency independent. 2D-SFG spectroscopy The different static SFG spectrum and surface vibrational dynamics of aqueous solutions of NaCl and NaI in comparison with pure water already qualitatively indicate that both chloride and iodide ions are surface active. In the following, we will show how the density of interfacial ions can be quantified using two-dimensional (2D)-SFG spectroscopy. In these experiments, the excitation pulse is scanned across the hydrogen-bonded part of the SFG spectrum, with excitation frequencies indicated by the dashed lines in Fig. 1 . By combining transient spectra such as depicted in Fig. 2a for different excitation frequencies and subtracting the thermal and oscillatory contributions signals, we obtain 2D-SFG spectra, as shown in Fig. 3 . These spectra present the SFG intensity as a function of excitation (horizontal axis) and detection frequency (vertical axis). In this experiment, a vibrational mode is excited at a particular frequency, and the effect of this excitation is probed over a wide range of detection frequencies. If the OD modes are uncoupled, there will only be a transient SFG signal at detection frequencies that correspond to the SFG spectrum of the excited OD mode. As a result, the 2D-SFG spectrum will be tilted with respect to the excitation frequency axis (see Fig. 3a,d ), provided that the OD modes at the surface possess a certain heterogeneity. As such, the slope of the 2D-SFG response at zero delay constitutes a measure of the heterogeneity of the interface. 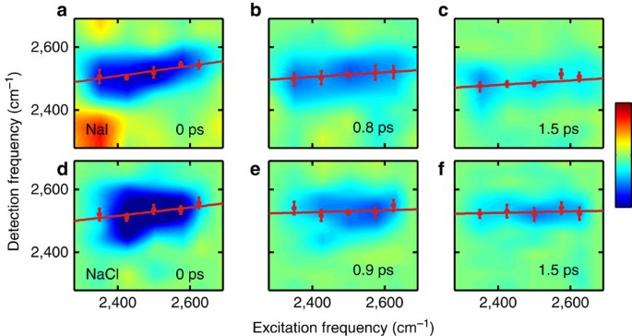Figure 3: Time-dependent 2D-SFG spectra. SFG intensity as a function of excitation and detection frequency for 3 M NaI (a–c) and NaCl (d–f) solutions recorded at different delay times between the excitation and detection pulses. Colorbar scale runs from −0.2 to +0.2. Points indicate central position of a Gaussian function fitted for each excitation frequency, whereas lines indicate their linear regressions. The error bars indicate central positions of the Gaussian fits for which theχ2value doubles. Figure 3: Time-dependent 2D-SFG spectra. SFG intensity as a function of excitation and detection frequency for 3 M NaI ( a – c ) and NaCl ( d – f ) solutions recorded at different delay times between the excitation and detection pulses. Colorbar scale runs from −0.2 to +0.2. Points indicate central position of a Gaussian function fitted for each excitation frequency, whereas lines indicate their linear regressions. The error bars indicate central positions of the Gaussian fits for which the χ 2 value doubles. Full size image We observe that the initial slope is smaller for the two studied salt solutions than for pure D 2 O [2] . With increasing delay time, the 2D-SFG response becomes increasingly horizontal ( Fig. 3c,f ). The time evolution of the slope of the 2D-SFG response reflects the decay of the frequency–frequency correlation function, that is, the loss of the spectral heterogeneity, due to spectral diffusion: OD groups initially excited at one frequency, change their frequency in the course of time. This may result from either structural relaxation or intermolecular resonant energy transfer [29] , [30] , [31] , [32] . For water at the water/air interface, we have previously found resonant Förster energy transfer to dominate the decay of the frequency–frequency correlation function [2] . The same mechanism is expected to dominate the spectral relaxation of salt solutions, since structural relaxation for water hydrating ions is slower than that of pure water [25] , [26] , [33] . To quantify the time-dependent slope of the 2D-SFG spectra, we determine the maxima (by fitting a Gaussian profile) of the SFG response at each excitation wavelength, for each time delay (red circles in Fig. 3 ). Subsequently, we fit a line (red lines in Fig. 3 ) to the central positions of the Gaussian profiles (weighted with their integrated intensities). 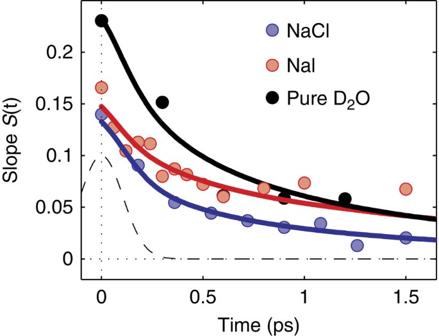Figure 4: Slope of the 2D-SFG response as a function of time. Points indicate slope values for three molar salt solutions (red and blue) and pure water (black), whereas lines depict calculations using the intermolecular energy transfer model, described in detail in the main text. The fitted curves were convoluted with the instrument response function (dashed line). Slope dynamics of the 2D-SFG response Figure 4 depicts the time-dependent slope values of the 2D-SFG spectra of solutions of 3 M NaI and 3 M NaCl in D 2 O, and of pure D 2 O, for comparison [2] . The slopes of the salt solutions have a smaller initial value and show a significantly slower decay than the slope of pure D 2 O. The slope of the iodide solution shows the slowest decay. The smaller initial slope values of the salt solutions indicate that, despite the presence of ions, the environment of the water molecules is spectrally less heterogeneous than for pure D 2 O. The slower decay of the slopes for the salt solutions means that resonant energy transfer is slower at the surface of a concentrated salt solution than at the surface of pure water. The energy transfer rate depends very strongly on the average intermolecular distance between water molecules. The slowing down of the resonant vibrational energy transfer thus shows that the average distance between OD groups is larger at the surface of salt solutions than at the surface of pure D 2 O. The presence of ions at the surface serves to dilute the water, and thereby increases the average distance between the OD groups. Figure 4: Slope of the 2D-SFG response as a function of time. Points indicate slope values for three molar salt solutions (red and blue) and pure water (black), whereas lines depict calculations using the intermolecular energy transfer model, described in detail in the main text. The fitted curves were convoluted with the instrument response function (dashed line). Full size image We can quantify the dilution effect using the previously derived formula describing resonant Förster energy transfer at the interface [2] : where N A is Avogadro’s number, r 0 the distance over which the energy transfer occurs with 50% efficiency, and S 0 the initial slope. The dipole–dipole coupling strength is expressed by . We reference all r 0 values to the T 1 of 1.7 ps of the OD vibration of bulk HDO in H 2 O, thereby ensuring that r 0 forms a direct measure of the relative strength of the dipole–dipole couplings in the different solutions. This equation successfully describes the energy transfer for interfacial water of pure D 2 O, with r 0 :D 2 O=2.1 Å (see Methods and ref. 2 ). Minor corrections for the small changes in the transition dipole moment, absorption linewidths and slightly different refractive indices of salt solutions with respect to bulk D 2 O (see Methods) result in r 0:NaI =2.00±0.02 Å and r 0:NaCl =2.10±0.02 Å. Using these values for r 0 , we can determine C OD representing the concentration of OD groups taking part in the energy transfer. For pure D 2 O, the concentration of D 2 O molecules amounts to 55.3 mol l −1 , corresponding to a concentration of OD oscillators C OD =2 × 55.3=110.6 mol l −1 . We note that the derived concentration values represent concentrations that are averaged over the SFG probing depth (~6 Å). We fitted the value C OD to the slope dynamics of the ionic solutions using Equation 1. The results of the fits are represented by the solid lines in Fig. 4 . Evidently, the Förster model provides a very good description of the observed slope dynamics. We find the water concentration at the interface to be C OD =103±10 mol l −1 and C OD =83±10 mol l −1 for NaCl and NaI, respectively. For both solutions, the extracted C OD is thus significantly lower than that of bulk water C OD =110.6 (55.3 mol l −1 D 2 O molecules). The reduction in C OD can be explained by the presence of the halide anions. From the extracted C OD values, it follows that ~4 and ~14 moles of water, from the surface of the NaCl and NaI solutions respectively, have been replaced by ions. These numbers of water molecules can be directly converted into a surface anion concentration using the sizes of a water molecule and the anions. The volume of a single water molecule corresponds to a sphere with a radius of 2.0 Å, while the chloride and iodide anions have radii of 1.81 and 2.2 Å, respectively [34] . Given that no ion pairing occurs for the studied salts [35] , [36] , that the volume taken by a bare Na + ion is ~6/~11 times smaller than that of a bare Cl − /I − ion (ionic radius of sodium: 1.02 Å), and that the sodium ions are hardly present in the probed surface layer [11] , [15] , [16] , [24] , we neglect the effect of the cation in calculating interfacial concentrations. We derive an effective interfacial concentration of chloride of (2.0/1.81) 3 × 4=5.5 M, and of iodide of (2.0/2.2) 3 × 14=10.5 M. These extracted interfacial anion concentrations are approximately (~5.5 M versus ~3 M) and times higher (~10.5 M versus ~3 M) than the concentrations in the bulk solution, where the errors reflect the uncertainty in r 0 for the different samples, and in the corrections to r 0 for the two solutions. In summary, we have measured the rate of resonant vibrational energy transfer between D 2 O molecules at the surface of solutions of NaCl and NaI in D 2 O. The measured rate of energy transfer serves to quantify the effective water concentration and the ion concentration at the surface. We find that the concentration of chloride is (~5.5 M versus ~3 M) and of iodide is times higher (~10.5 M versus ~3 M) at the surface than in bulk. Our findings are of fundamental importance for processes in atmospheric chemistry. Specifically, it has recently been shown that significant levels of atmospheric iodine originate from the interfacial chemistry at the oceans interfaces, and is associated with ozone reduction [5] . The quantitative modelling of these processes requires detailed knowledge of the surface propensity of the different ions present in sea water. Experimental setup The vibrational dynamics of aqueous salt solutions/air interfaces has been studied using time-resolved 2D- SFG spectroscopy (2D-SFG). In the experiment, we use an IR-pump/SFG-probe scheme, where the pump pulses are spectrally narrow (~100 cm −1 ), and tuned across the absorption band of water. For the detection process, broadband mid-IR and narrow band VIS upconversion pulses are mixed at the interface to generate a conventional SFG signal. These pulses are generated by frequency conversion processes that are pumped with the 800 nm pulses derived from a high energy Ti:Sapphire amplifier system. This system comprises a regenerative amplifier (‘Legend Duo’, Coherent) that delivers 40 fs pulses with a pulse energy of 6 mJ and a repetition rate of 1 kHz. We use approximately 4.5 mJ to pump an optical parametric amplifier (HE-TOPAS, Light Conversion). The produced signal and idler pulses are used in a difference frequency mixing process in a silver gallium disulphide (AgGaS 2 ) crystal resulting in 80 μJ pulses, tunable around a central wavelength of ~4000, nm (~2500, cm −1 ), a pulse duration of ~60 fs full width at half maximum (FWHM), and a spectral bandwidth of ~400 cm −1 (FWHM). This bandwidth is sufficient to cover the whole vibrational band of water. The remaining 1.5 mJ of 800 nm pulses travel through an etalon (SLS) yielding narrow band pulses (15 cm −1 FWHM), which are used in the SFG process. The high-intensity and narrow band pump pulses are generated in an independent parametric conversion process in which we use the residual 800 nm and idler pulses from the TOPAS. The idler pulses are doubled in a β-barium borate crystal, resulting in pulses with a central wavelength of ~1000, nm. Subsequently, the doubled idler and 800 nm pulses are combined in a difference frequency mixing process in a LiNbO 3 crystal. This results in ~45 μJ pulses, with a central wavelength between 2100 and 2900 cm −1 and a pulse duration less than 200 fs. The bandwidth of the pump pulses is typically 100 cm −1 , and always between 80 and 150 cm −1 . Both pump and probe pulses are continuously monitored with a frequency resolved IR detection setup consisting of an ORIEL monochromator and a 2 × 32 pixels, mercury–cadmium–telluride array detector. In the experiment, the pump frequency is scanned across the absorption band of water. For each excitation frequency, the time delay between the pump and probe-pair pulses is varied using a mechanical delay line, and a series of sum frequency spectra at different delay times are recorded. The IR pump, probe and VIS beams with energies of typically 12, 6.5 and 10 μJ per pulse span a vertical plane and have respective incident angles of 56°/40°/70° with respect to the surface normal. The polarization of the SFG/VIS/IR beam was controlled using λ /2 plates and set to S/S/P in all experiments, respectively. The polarization of the pump pulses was P. The third order cross correlation between the pump, the probe and the VIS pulses generated at the samples surface is used to optimize the SFG signal and to determine the time overlap between the excitation and probe-pair pulses. Sample preparation D 2 O (Cambridge Isotope Laboratories. Inc., 99.96 atom %D) was used as received (pD=~5.5). NaCl, NaI and sodium thiosulfate (Na 2 S 2 O 3 ) were purchased from Sigma Aldrich. NaCl and NaI salts are used to prepare 3 M solutions in D 2 O. NaCl was baked at around 500 °C for more than 6 h in order to remove any organic impurities. We added 50 mM of sodium thiosulfate to the NaI solution to prevent the oxidation reaction of iodide ions. In the experiment, we use heavy water (D 2 O) rather than normal water (H 2 O) for two reasons: firstly, heavy water possesses a longer vibrational lifetime allowing for a longer observation window for the vibrational energy transfer process, and, secondly, the OD stretch mode has a narrower linewidth allowing the probing of the complete SFG spectrum without tuning the IR frequency. The Teflon sample trough was cleaned with piranha solution (3:1 volume ratio of sulphuric acid and 30% hydrogen peroxide solution) and continuously rotated during the experiment to avoid steady state heat accumulation in the sample. We use an automatic feedback loop to control the vertical sample position, compensating for water evaporation and to ensure that the concentration of the sample does not change throughout the experiment. The setup was enclosed and flushed with N 2 gas in order to remove spectral distortions originating from the CO 2 absorption in the air. All experiments have been performed several times to ensure reproducibility. Correction for heating and oscillatory signals The population dynamics N ( t ) of each state and corresponding spectral signatures σ ( ω, ω exc ) are determined by fitting the data to a kinetic model formed by the following set of rate equations: The phase ( φ ), period and damping rate ( k damping ) of the oscillatory signals were determined by fitting a single dataset (2500, cm −1 excitation), integrated over 100 cm −1 around the central frequency of 2500, cm −1 . We will report on these oscillations in a forthcoming publication (Hsieh, C. S., Piatkowski, L., Bakker, H. J. and Bonn, M., manuscript in preparation). We fit the datasets for all excitation frequencies simultaneously, keeping the relaxation rate k 1 as the global parameter. Results of the global fit for the NaI solution at 2500, cm −1 excitation, including spectra of the three states and corresponding population dynamics, are shown in Supplementary Fig. 1 . Förster radius r 0 The extracted value of the OD oscillators participating in the Förster energy transfer C OD depends on the value of the Förster radius r 0 . We thus have to correct the value for r 0 obtained for the pure D 2 O/air interface for the change in cross section and linewidth of the OD stretch absorption bands. We correct here a mistake due to a programming error in ref. 2 : the value of the Förster radius r 0 =2.1 Å for pure D 2 O/air interface, rather than the value r 0 =2.4 Å reported in ref. 2 . We note that this does not affect any of the conclusions drawn in ref. 2 . The rate of energy transfer between the same type of oscillators is defined as , where σ is the absorption cross section, R is the distance between the oscillators and the integral of the squared lineshape g(ν) reflects the spectral overlap between the donor–acceptor pairs [37] . Under the assumption that the orientation of the oscillators is random, the rate of the energy transfer between donor and acceptor can be expressed as . Comparing the two expressions, it becomes clear that any change in the absorption cross section and/or absorption lineshape will affect the value of the Förster radius: . In principle, r 0 will also change if T 1 changes. However, we reference all r 0 values to the same value of T 1 of 1.7 ps of the OD vibration of bulk HDO in H 2 O, in order to retain the value of r 0 as a good measure for the strength of the dipole–dipole coupling in the different solutions. Finally, the Förster radius r 0 depends on the refractive index of the medium intervening with the energy transfer as . Since the refractive indices of salt solutions are somewhat higher than the refractive index of bulk D 2 O, we take this into account when correcting the Förster radius. The corrected Förster radius for water molecules in salt solution can be directly obtained from: The ratio of the cross sections being defined as: where and are the frequency-integrated linear absorption spectra of the salt solutions and pure D 2 O, respectively (see Supplementary Fig. 2 ). and are the effective concentrations of D 2 O molecules in salt solution and pure D 2 O, respectively. Using the densities of salt solutions d NaI =1.4474 (g ml −1 ) [38] and d NaCl =1.208 (g ml −1 ) [39] , we find 51.3 M and 51.5 M of D 2 O in 3 M NaI and NaCl solutions respectively. Pure D 2 O contains 55.3 M of D 2 O molecules. Integrals of the measured linear absorption (ATR) spectra (see Supplementary Fig. 2 ) amount to (a.u. ), (a.u.) and (a.u.). ATR spectra of salt solutions are sensitive to the water content and the refractive index of the solution. Direct comparison of the experimental ATR spectra requires thus a correction for the density of water and the refractive index of measured solutions, according to the formula derived by Max et al . [40] : Corrected linear absorption integrals amount to (a.u.) and (a.u.). Using equation (2), we thus find that and . The linear absorption spectra of salt solutions are narrower than the linear absorption spectrum of pure D 2 O (measured at FWHM) by approximately 5%, implying that the self-overlap of the absorption band of OD oscillators in salt solutions is ~1.05 larger compared with self-overlap of the OD oscillators in pure water: . The refractive index of heavy water (measured at 1.6 μm) amounts to (ref. 41 ). The refractive indices of the salt solutions are calculated using n = n 0 + Cn 1 , where n 0 is the refractive index of the solvent, C is the concentration of the solute and n 1 is a salt specific correction factor [42] . The thus calculated refractive indices of the bulk salt solutions are and . Due to the lower density of the interfacial layer and the vicinity of another dielectric medium (air), we need to determine the effective interfacial refractive indices. These are calculated with the equation presented by Zhuang et al . [43] Since the refractive indices of the salt solutions are dependent on the interfacial ion concentration that we intend to extract from the fit to the data, we use here an iterative approach: first we assume an interfacial ion concentration C ; then calculate the effective interfacial refractive index; correct the Förster radius r 0 and finally perform the fit to the data. We repeat these steps until the extracted interfacial anion concentration matches the one used for the correction. We reach convergence at a concentration of 10 M for the NaI solution and at a concentration of 5 M for the NaCl solution. For these concentrations, the effective interfacial refractive indices are and . Substituting all the above mentioned numbers into Equation 5, we find that the following corrected Förster radii for the salt solutions and Instrument response We convolute the Förster formula with the system response function, which has been determined from the time-dependent third-order cross correlation function of the pump, probe and VIS pulses (denoted with the dashed line in Fig. 4 ), in order to account for the non-zero durations of the IR light pulses. In the fit of the Förster formula to the data, the data points are weighted with the total intensity of the SFG bleach signal at the corresponding delay time. How to cite this article: Piatkowski, L. et al . Extreme surface propensity of halide ions in water. Nat. Commun. 5:4083 doi: 10.1038/ncomms5083 (2014).